Dynamics of an initially spherical bubble rising in quiescent liquid The beauty and complexity of the shapes and dynamics of bubbles rising in liquid have fascinated scientists for centuries. Here we perform simulations on an initially spherical bubble starting from rest. We report that the dynamics is fully three-dimensional, and provide a broad canvas of behaviour patterns. Our phase plot in the Galilei–Eötvös plane shows five distinct regimes with sharply defined boundaries. Two symmetry-loss regimes are found: one with minor asymmetry restricted to a flapping skirt; and another with marked shape evolution. A perfect correlation between large shape asymmetry and path instability is established. In regimes corresponding to peripheral breakup and toroid formation, the dynamics is unsteady. A new kind of breakup, into a bulb-shaped bubble and a few satellite drops is found at low Morton numbers. The findings are of fundamental and practical relevance. It is hoped that experimenters will be motivated to check our predictions. The motion of a gas bubble rising due to gravity in a liquid has been studied from many centuries ago and continues to be a problem of great interest today. Interestingly, the fact that this dynamics is three-dimensional (3D) was first documented by Leonardo Da Vinci in the 1500s. In the past several decades, thousands of published works have attempted to fit various regimes of the bubble motion into simple models. Bubble dynamics is of huge importance in heat and mass transfer, in natural phenomena like aerosol transfer from sea, oxygen dissolution in lakes due to rain and electrification of atmosphere by sea bubbles [1] , in bubble column reactors, in the petroleum industry, for the flow of foams and suspensions and in carbon sequestration [2] , to name just a few. The number of parameters, the nonlinearity and the fully 3D nature of the problem makes it vast and daunting. This problem is completely described by four non-dimensional parameters, see for example, ref. 3 : the Galilei number (Ga), the Eötvös number (Eo), the density ratio ρ r and the viscosity ratio μ r (see below). A rising bubble may never display a steady terminal velocity, and even if it does, the terminal velocity is not known a priori , so the Galilei and Eötvös numbers are better suited to describe the dynamics of rising bubbles rather than the Reynolds and Weber numbers (which contain the terminal velocity). We will also make use of the Morton number, Mo ≡ Eo 3 /Ga 4 , which is a constant for a given liquid–gas system. We now discuss select earlier studies. While most earlier computational studies have been axisymmetric or two-dimensional (2D), several 3D simulations have been done as well, see for example, refs 4 , 5 , 6 , 7 , 8 , 9 , 10 , 11 , 12 . A remarkable set of papers [5] , [6] , [13] , [14] , [15] study bubbly flows in which the interaction between the flow and a large number of bubbles is studied. In particular, turbulent flows can be significantly affected by bubbliness. These studies typically used one or two sets of Eötvös number and Galilei number. There have also been several studies in which the computational techniques needed to resolve this complicated problem have been perfected [7] , [8] , [9] , [11] , [12] , [16] . Furthermore, ref. 17 reported a numerical technique that combines volume of fluid and level-set methods and limits the interface to three computational cells. It is remarkable in its relative simplicity in the extension from 2D to 3D. This problem has attracted a large number of experimental studies as well, see for example, refs 18 , 19 . A library of bubble shapes is available, including skirted, spherical cap and oscillatory and non-oscillatory oblate ellipsoidal. Approximate boundaries between the regimes where each shape is displayed are available in refs 20 , 21 for unbroken bubbles. The boundaries we obtain between different regimes for unbroken bubbles are in broad agreement with these experimental studies. In experiments on larger bubbles, the shapes at release are designed to be far from spherical. Second, experiments that give a detailed description of the flow field are few, and accurate shape measurements are seldom available. An important point is that bubble shapes and dynamics are significantly dependent on initial conditions at release, which are difficult to control in experiments. One of our objectives is to standardize the initial conditions, a luxury not easily available to experimenters! A curious phenomenon, the path instability, has been the subject of a host of experimental [22] , [23] , [24] , [25] , numerical [26] , [27] and analytical [28] , [29] studies. This is the name given to the tendency of the bubble, under certain conditions, to adopt a spiral or zigzagging path rather than a straight one. After Prosperetti (2004) discovered it in the books of Leonardo Da Vinci, he termed the path instability as Leonardo's paradox, since it was not known then why an initially axisymmetric bubble would take up a spiral or zigzag path. We will demonstrate that path and shape symmetry are intimately connected, but only the former has been measured experimentally. It is not easy to measure the evolving bubble shape [24] and flow field accurately in this highly 3D regime. Most of the workers embarking on this study find it satisfactory to investigate the effect of initial bubble diameter on the rising dynamics, and no experimental investigations are available to our knowledge which study the effects of just the surface tension or viscosity of water on the bubble rise. We mention one study [19] here where the effect of surfactant concentration on the oscillatory motion of bubbles is evaluated. The path instability of bubbles was obtained by numerical stability analysis of a fixed axisymmetric bubble shape by refs 26 , 27 ; these will be discussed below. An interesting numerical study of ref. 30 shows hairpin vortices in the wake of an initially zigzagging bubble. A vast majority of the earlier experimental and theoretical studies have had one of the following goals: to obtain the rise velocity, to evaluate the path instability, to understand bubbly flows, to make quantitative estimates for particular industrial applications, or to derive models for estimating different bubble parameters. Most of these restrict themselves to only a few Ga or Eo. Our study, in contrast, is focussed on the dynamics of a single bubble. Starting from the initial condition of a spherical stationary bubble, we are interested in delineating the physics that can happen. We cover a range of several decades in the relevant parameters. We study bubbles rising due to buoyancy in a far denser and more viscous fluid. We show that as the size of the bubble is increased, the dynamics goes through three abrupt transitions from one known class of shapes to another. A small bubble will attain an axially symmetric equilibrium shape dictated by gravity and surface tension, and travel vertically upwards at a terminal velocity thereafter. A bubble larger than a first critical size loses axial symmetry. We show that this can happen in two ways. Beyond the next critical size, it breaks up into a spherical cap and many satellite bubbles, and remarkably, the cap regains axial symmetry. Finally, a large bubble will prefer not to breakup initially, but will change topologically to become an annular doughnut-like structure, which is perfectly axisymmetric. The rising bubble phase plot We begin by defining the Galilei number , which is a ratio of the gravitational force to the viscous force; the Eötvös number Eo(≡ ρ o gR 2 / σ ), which is a ratio of the gravitational force to the surface tension force; the density ratio ρ r (≡ ρ i / ρ o ), and the viscosity ratio μ r ( ≡ μ i / μ o ), where g , R and σ , respectively, are the gravitational acceleration, initial radius of the spherical bubble and the surface tension coefficient for the pair of fluids considered; ρ i , μ i and ρ o , μ o are the density and dynamic viscosity of the dispersed and the continuous phases, respectively. In the present study, ρ r and μ r are fixed at 10 −3 and 10 −2 , respectively. 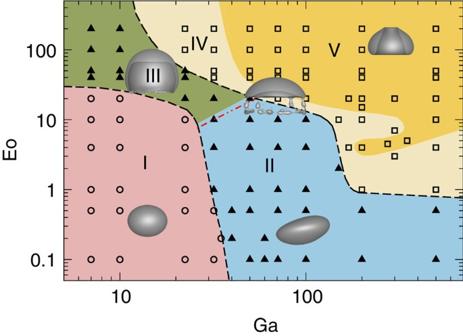Figure 1: Different regimes of bubble shape and behaviour. The different regions are: axisymmetric (circle); asymmetric (solid triangle); and breakup (square). The axisymmetric regime is called region I. The two colours within the asymmetric regime represent non-oscillatory region II (shown in green), and oscillatory region III (blue) dynamics. The two colours within the breakup regime represent the peripheral breakup region IV (light yellow), and the central breakup region V (darker yellow). The red dash–dotted line is the Mo=10−3line, above which oscillatory motion is not observed in experiments in refs21,22. Typical bubble shapes in each region are shown. In this and similar figures below, the bubble shapes have been made translucent to enable the reader to get a view of the internal shape. Figure 1 represents a summary of what happens to an initially spherical bubble rising under gravity in a liquid. A range of ratios of gravitational, viscous and surface tension forces have been simulated (in about 130 simulations). Several features emerge from this phase plot, which is divided into five regions. Region I, at low Eötvös and Galilei numbers, is shown in pink. In this region, surface tension is high and gravity is low, so it is understandable that the bubble retains its integrity. It attains a constant ellipsoidal shape, of which a typical example is shown in the figure in that region, and takes on a terminal velocity going straight upwards. The bubble is axisymmetric in this region. Region II, at high Eötvös numbers and low Galilei numbers, is demarcated in green colour. The bubble here has two distinct features, an axisymmetric cap with a thin skirt trailing the main body of bubble. The skirt displays small departures from axisymmetry in the form of waves, for example, a wavenumber 4 mode is barely discernible in the typical shape shown. Bubbles in this region travel upwards in a vertical line as well, and practically attain a terminal velocity after the initial transients and display shape changes only in the skirt region. The extreme thinness, in parts, of the skirt presents a great challenge for numerical analysis and a detailed study of this region is left for the future. Region III, depicted in blue colour, occupies lower Eötvös and higher Galilei numbers. Here surface tension and inertial forces are both significant, and of the same order. Bubbles display strong deviations from axisymmetry in this region, at relatively early times, and rise in a zigzag or a spiral manner. Bubbles remain integral, but their shapes change with time. Region IV is shown in light yellow colour, and region V is in dark yellow. The bubble, faced with higher gravity and relatively weak surface tension, breaks up or undergoes a change of topology in these regions. Remarkably, the dynamics may be described well as axisymmetric up almost to the breakup. Region IV is a narrow region that may be described roughly as having a moderate value of the product Ga–Eo. At low Ga and high Eo (that is, high Morton number) the bubble in this regime breaks into a large axisymmetric spherical cap and several small satellite bubbles in the cap's wake. We term this a peripheral breakup, since it involves a pinch-off of a skirt region of the kind seen in region II. For high Ga and low Eo (that is, lower Mo) a new breakup dynamics is observed, not hitherto described to our knowledge, which is discussed below. Significant among the results is the fact that in region IV, after breakup axisymmetry is regained and the final spherical cap bubble attains a constant shape and terminal velocity. Finally, the bubbles shown is region V are under the action of high inertial force and low surface tension force. A qualitatively different kind of dynamics is seen here. A dimple formation in the bottom centre leads to a change of topology: to a doughnut-like or toroidal shape as seen in the figure. Close to the boundary of region IV, the change of topology may be accompanied by an ejection of small satellite bubbles. As Ga and Eo are increased further in this region, a perfectly axisymmetric change of topology of the whole bubble is observed. Unlike in the other regions, this new shape is not permanent. It eventually loses symmetry and evolves into multiple bubble fragments. The boundaries between the five regions are easy to distinguish because the time evolution is qualitatively different on either side. Details of how a bubble is assigned to a particular region are provided in the Methods section. Moreover the sum of the kinetic and surface energies usually goes to a maximum at the transition between two regions, and falls on either side. This is exemplified in the Supplementary Fig. 7 . Figure 1: Different regimes of bubble shape and behaviour. The different regions are: axisymmetric (circle); asymmetric (solid triangle); and breakup (square). The axisymmetric regime is called region I. The two colours within the asymmetric regime represent non-oscillatory region II (shown in green), and oscillatory region III (blue) dynamics. The two colours within the breakup regime represent the peripheral breakup region IV (light yellow), and the central breakup region V (darker yellow). The red dash–dotted line is the Mo=10 −3 line, above which oscillatory motion is not observed in experiments in refs 21 , 22 . Typical bubble shapes in each region are shown. In this and similar figures below, the bubble shapes have been made translucent to enable the reader to get a view of the internal shape. Full size image We had mentioned the Morton number above, defined as Mo=Eo 3 /Ga 4 . This combination deserves a separate name because it depends only on the fluid properties and not on the bubble size. Air bubbles in a particular fluid at a particular temperature will lie on constant Morton number lines, which are straight lines in the log–log phase plot. The red dashed line in Fig. 1 corresponds to a Morton number of 10 −3 , which is the Morton number mentioned in numerous experiments, see for example, refs 21 , 22 below which spiralling and zigzagging trajectories are seen. Note that the boundary between regions II and III, that is, between straight and zigzagging trajectories, in our simulations lies very close to this. The lines of constant Morton number corresponding to some common liquids at different temperatures are shown in Fig. 2 . Since we have used very small viscosity and density ratios, our results apply to various air–liquid systems. In the examples given, the liquid densities are not far from water, and we know from refs 31 , 32 that the dynamics is insensitive to viscosity ratio for small μ r . Moving upwards and to the right on a given line, the bubble size increases and typical bubble sizes are indicated in the figure. We see that our results apply to a range of liquids in which an estimate of bubble motion may be desired, for instance crude oil, water at different temperatures and cooking oils. A 1-mm radius bubble in water at room temperature will execute spiral or zigzag motion whereas a 20-mm bubble in honey will develop a skirt but move upwards in a straight line. It is to be noted that only in Fig. 2 we mention dimensional radii for particular liquids, whereas all the other results are presented in non-dimensional form. 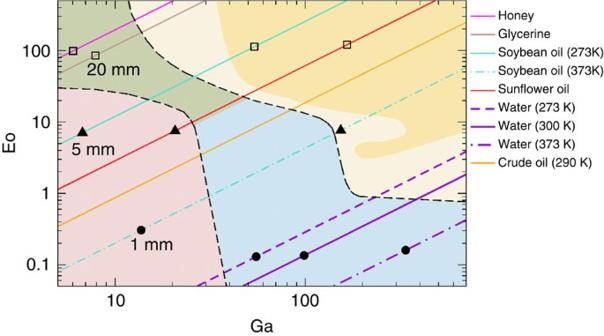Figure 2: Dynamics expected for bubbles in different liquids. Constant Morton number lines, each corresponding to a different liquid, are overlayed on the phase plot to demonstrate that our transitions can be easily encountered and tested in commonly found liquids. The initial radius of the air bubble increases from left to right on a given line. Circles, triangles and squares represent air bubbles of 1, 5 and 20 mm radii, respectively. Figure 2: Dynamics expected for bubbles in different liquids. Constant Morton number lines, each corresponding to a different liquid, are overlayed on the phase plot to demonstrate that our transitions can be easily encountered and tested in commonly found liquids. The initial radius of the air bubble increases from left to right on a given line. Circles, triangles and squares represent air bubbles of 1, 5 and 20 mm radii, respectively. Full size image We had recently shown ref. 3 that a bubble is more likely to lose its original topology to attain a doughnut shape at high inertia and low surface tension, whereas a drop under the same Eötvös and Galilee numbers would tend to break into several drops. We predicted that non-Boussinesq effects are qualitatively different in drops and bubbles, since highly vortical regions are stable when situated within the lighter fluid. The present 3D simulations are a confirmation of this physics. Path instability and shape asymmetry Two portions of our phase space have received particular attention earlier. The first, which we have spoken of earlier, is the onset of zigzagging motion, famously referred to as the path instability. Ryskin and Leal [33] and many other studies believed the path instability to occur due to vortex shedding from the bubble. Indeed, in the motion of solid objects through fluid this is the only way in which one can get a path, which is not unidirectional. Magnaudet and Mougin [26] assumed the bubble to be ellipsoidal in shape, and studied a constant velocity flow past such a bubble to obtain the instability of its wake. The bubble shape and position were held fixed during the simulation. An asymmetric wake was taken to be indicative of the onset of zigzagging motion. Cano-Lozano et al. [27] repeated a similar analysis, but on a realistic bubble shape, which they obtained from axisymmetric numerical simulations. The bubble was held in a constant velocity inlet flow equal to the terminal velocity obtained in their simulations for the axisymmetric shape. Wake instabilities were the investigated from a 3D simulation of this fixed bubble. We find that this simplified method yields a good qualitative estimate of the onset of zigzagging motion at low inertia. A comparison with our more exact 3D simulations is shown in Fig. 3 , where quantitative discrepancies are noticed, especially for large inertia, that is, Ga>50. Also given in this figure is a comparison with the very recent results of ref. 12 . For five different pairs of Ga and Eo, the dynamics predicted by these authors may be seen to be confirmed by present results. While we did not distinguish our shapes into spherical and ellipsoidal, we note that the boundary provided by ref. 34 , also shown in this figure, between spherical and non-spherical shapes, is consistent with our findings. The line falls well within our regions I and II where we have ellipsoidal drops, and in region II lies close to the minimum Eo of our computations. 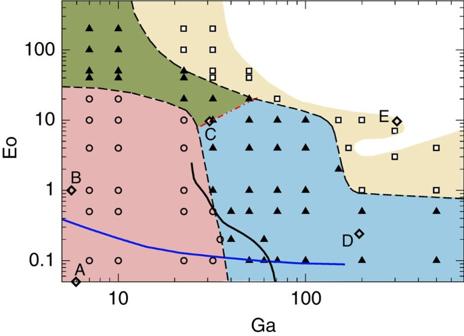Figure 3: Agreement and contrast between present and previous results for different flow regimes. Comparison between the onset of asymmetric bubble motion obtained in the numerical stability analysis of Cano-Lozanoet al.27(solid black line), and the present boundary between regions I and II. Also given in this figure are five different conditions (diamond symbols) studied by Baltussenet al.12The dynamics they obtain are as follows: A—Spherical, B—Ellipsoidal, C—Boundary between skirted and ellipsoidal, D—Wobbling and E—Peripheral breakup. The correspondence between present results and12is excellent. Graceet al.34obtained spherical bubbles below the solid blue line shown. Figure 3: Agreement and contrast between present and previous results for different flow regimes. Comparison between the onset of asymmetric bubble motion obtained in the numerical stability analysis of Cano-Lozano et al. [27] (solid black line), and the present boundary between regions I and II. Also given in this figure are five different conditions (diamond symbols) studied by Baltussen et al. [12] The dynamics they obtain are as follows: A—Spherical, B—Ellipsoidal, C—Boundary between skirted and ellipsoidal, D—Wobbling and E—Peripheral breakup. The correspondence between present results and [12] is excellent. Grace et al. [34] obtained spherical bubbles below the solid blue line shown. Full size image A point to note is that unlike solid spheres, departures from vertical motion in a bubble can be caused either by shape asymmetries, or unsteady vortex shedding or both. The stability analyses discussed above take account only of the latter, whereas experiments, for example, those of ref. 35 in clean water found a regime of path instability where no vortex shedding was expected. In fact a recent analytical study [29] , attempts to explain that vortex shedding is the effect, rather than a cause of the path instability in rising bubbles. Without a statement as to cause and effect, we expect an intimate connection between loss of symmetry and loss of a straight trajectory. Any asymmetry in the plane perpendicular to gravity should result in an imbalance of planar forces. Similarly any asymmetry in the planar forces, due to vortex shedding or otherwise, should result in shape asymmetry. In accordance with these expectations, we find that path instability and shape asymmetry go hand in hand, so the onset of path instability is just the boundary between regions I and III. Not just the onset, but the entire region III, where the bubble shape is strongly non-axisymmetric, coincides with the regime where path instability is displayed. 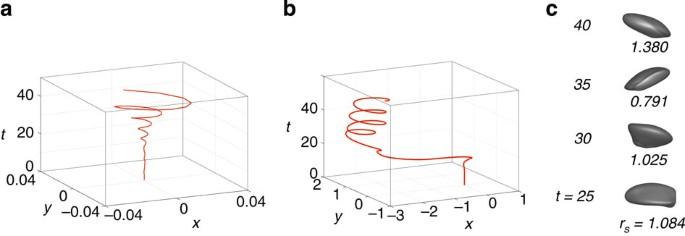Figure 4: Trajectory and shapes of typical region III bubbles. The trajectory of the bubble centroid for (a) Ga=70.7, Eo=10 and (b) Ga=100, Eo=4, and (c) shape evolution of bubble corresponding to the latter case. Inc, the radial distance of the centre of gravity (rs) of the bubble measured in the horizontal plane from the original location is shown below the shapes at each time. Figure 4 shows the trajectory, and the shape of a typical bubble in this region at different times. A helical-like motion is executed in the cases shown, while the shape is continuously changing. The bubble does not adopt a standard geometry. Incidentally, in several of the simulations, the centre of the helix does not coincide with the original location in the horizontal plane. Nor are the windings of the helix periodic or regular. Most trajectories in this regime are indicative of chaotic dynamics. We also obtain trajectories resembling widening spirals, or those which execute a zigzag motion with the centroid lying close to some vertical plane and there seems to be no particular region in the Ga–Eo plane where one or the other dominates. Zigzag and helical motion is accompanied by oscillations in the vertical velocity as well, so the bubble alternately speeds up and slows down on its way. An example is seen in the vertical velocity plot of Fig. 5a . Two kinds of oscillatory behaviour in the velocity are clearly visible in the figure, one with increasing oscillations at early times and one with a different character at later times. At later times the dynamics is more erratic, but amplitudes of variation are lower. In the first part, vorticity is generated in the wake but remains vertically aligned and attached to the bubble. At time t >14 the drop begins to display zigzag motion (see Fig. 5b ). The wake now consists of a pair of counter-rotating two-threaded vortices, often considered to be a first sign of path instability [26] . This is soon followed by shedding of the vortices, which begins at t >20. We find that the onset of the second type of unsteadiness may be attributed to the start of the vortex shedding off the bubble surface. The vertical component of vorticity in this regime is shown in Fig. 5c . In some cases we find resemblences to the hairpin vortices of ref. 30 . The manner in which the shape of the bubble evolves during this process is shown in Fig. 5d . The correspondence between asymmetry in shape and the path instability is obvious. A few animations are available in http://www.iith.ac.in/~ksahu/bubble.html . Figure 4: Trajectory and shapes of typical region III bubbles. The trajectory of the bubble centroid for ( a ) Ga=70.7, Eo=10 and ( b ) Ga=100, Eo=4, and ( c ) shape evolution of bubble corresponding to the latter case. In c , the radial distance of the centre of gravity ( r s ) of the bubble measured in the horizontal plane from the original location is shown below the shapes at each time. 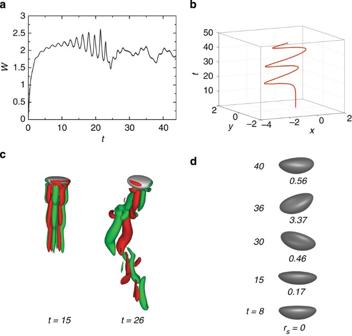Figure 5: Characteristics of a region III bubble of Ga=100 and Eo=0.5. (a) Oscillating axial velocity, with different behaviour at early and late times, (b) trajectory of the bubble centroid, (c) iso-surfaces of the vorticity component in thezdirection at timet=15 (ωz=±0.0007) and 26 (ωz=±0.006), (d) The evolution of the shape of the bubble. The radial distance of the centre of gravity (rs) of the bubble measured in the horizontal plane from the original location is shown below the shapes at each time. Full size image Figure 5: Characteristics of a region III bubble of Ga=100 and Eo=0.5. ( a ) Oscillating axial velocity, with different behaviour at early and late times, ( b ) trajectory of the bubble centroid, ( c ) iso-surfaces of the vorticity component in the z direction at time t =15 ( ω z =±0.0007) and 26 ( ω z =±0.006), ( d ) The evolution of the shape of the bubble. The radial distance of the centre of gravity ( r s ) of the bubble measured in the horizontal plane from the original location is shown below the shapes at each time. Full size image We bring out the importance of 3D simulations in Fig. 6 in regions III and IV. We saw that the path instability is deeply connected to shape asymmetries, so region III dynamics are inherently 3D. In region IV the breakup is not axisymmetric. We note that region I can be well obtained from 2D axisymmetric simulations. 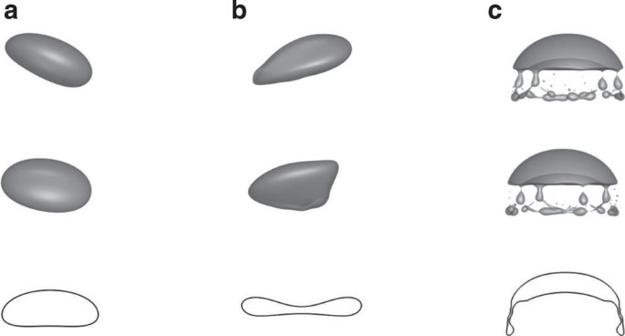Figure 6: Differences between 2D and 3D bubble shapes: (a) A region III bubble att=20 for Ga=100 and Eo=0.5, (b) att=30 for Ga=100 and Eo=4, again in reign III, and (c) a region IV bubble att=5 for Ga=70.71 and Eo=20. The second row shows the side view of the 3D shapes of bubbles rotated by 90 degrees about ther=0 axis with respect to the top row. Figure 6: Differences between 2D and 3D bubble shapes: ( a ) A region III bubble at t =20 for Ga=100 and Eo=0.5, ( b ) at t =30 for Ga=100 and Eo=4, again in reign III, and ( c ) a region IV bubble at t =5 for Ga=70.71 and Eo=20. The second row shows the side view of the 3D shapes of bubbles rotated by 90 degrees about the r =0 axis with respect to the top row. Full size image Breakup regimes We now examine the dynamics of bubbles destined for breakup, of regions IV and V. The contrast in bubble behaviour between these two regions is evident in Fig. 7 . At early times both bubbles are axisymmetric. The region IV bubble develops a skirt, in this case similar to the one seen in region II, with the difference that this skirt then breaks off in the form of satellite bubbles, leaving an axisymmetric spherical cap. The region V bubble was seen to first undergo a change in topology into a doughnut or toroid shape. Beyond time t =5, the toroid is subject to further instability and breaks into a number of droplets. Pedley [36] had predicted that a perfectly toroidal bubble of circular cross-section will undergo instability beyond a time t c . In our scales, the instability time of Pedley may be written as t c ~GaEo 1/2 f 3/2 , where f is the ratio of the inner radius of the toroid to the initial radius R . Given that our toroidal bubble has a cross section very far from circular, we expect instability to set in much sooner, and find breakup at times an order of magnitude lower than t c . In addition the history of the flow, including the vortex patterns, contribute to hastening instability. 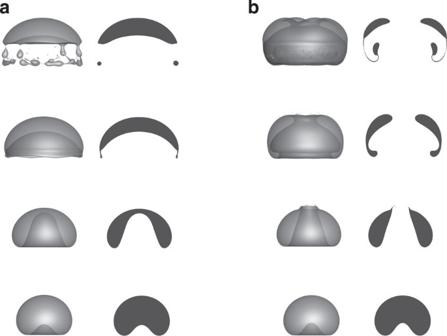Figure 7: Time evolution of bubbles exhibiting a peripheral and a central breakup. Three-dimensional and cross-sectional views of the bubble at various times (from bottom to top the dimensionless time is 1, 2, 4 and 5). (a) region IV, a bubble breaking into a spherical cap and several small satellite bubbles, Ga=70.7 and Eo=20, and (b) region V, a bubble changing in topology from dimpled ellipsoidal to toroidal, Ga=70.7 and Eo=200. Figure 7: Time evolution of bubbles exhibiting a peripheral and a central breakup. Three-dimensional and cross-sectional views of the bubble at various times (from bottom to top the dimensionless time is 1, 2, 4 and 5). ( a ) region IV, a bubble breaking into a spherical cap and several small satellite bubbles, Ga=70.7 and Eo=20, and ( b ) region V, a bubble changing in topology from dimpled ellipsoidal to toroidal, Ga=70.7 and Eo=200. Full size image Region IV bubbles show different breakup dynamics at higher inertia and surface tension (low Mo). For large Mo, a wide skirt was seen to form which then broke off into small bubbles, whereas for lower Mo values small bubbles are ejected from the rim of the bubble while it recovers from an initially elongated shape to the spherical cap shape. Bubbles of even lower Mo values, that is, at high inertia and surface tension, are subjected to strong vertical stretching giving rise to a far narrower skirt, which results in an ellipsoidal rather than a cap-like bubble and a small tail of satellite bubbles, as seen in Fig. 8 . This type of breakup has not been reported before, to our knowledge. 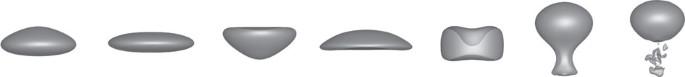Figure 8: A new breakup mode in region IV for Ga=500 and Eo=1. Bubble shapes are shown at dimensionless times (from left to right)t=2, 4, 6, 7, 8, 9 and 9.1). Figure 8: A new breakup mode in region IV for Ga=500 and Eo=1. Bubble shapes are shown at dimensionless times (from left to right) t =2, 4, 6, 7, 8, 9 and 9.1). Full size image Before breakup, departures from symmetry are small in region IV bubbles. Similarly region V bubbles are symmetric up to toroid formation. We may thus ask whether cap or toroid formation requires 3D. The transition from a spherical cap to a toroidal shape, as obtained by ref. 37 by means of axisymmetric computations are compared in Fig. 9 to our region IV—region V boundary, showing that the two trends agree qualitatively. The first difference between the axisymmetric and 3D simulations was seen in region IV in Fig. 6 . While the 2D simulations can only obtain breakup in the form of a ring that detaches from the spherical cap, our simulations enable the ejection of satellite bubbles. Another feature that the axisymmetric simulations will miss is the fact that the centre of gravity moves in the horizontal plane. Third, just below the lowest point given by ref. 37 , we obtain a protrusion of region V (seen in deep yellow in Fig. 9 ) pointing to the left and downwards in the Ga–Eo plane. The dynamics in this protrusion region is asymmetric, and seems to have been missed by other axisymmetric simulations. 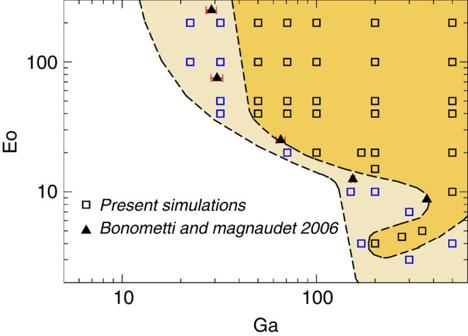Figure 9: Boundary between peripheral and central breakup regions. The light yellow and dark yellow colours represent the regions for peripheral and central breakup. The corresponding data points from the present numerical simulation are shown as blue and black squares, respectively. Results of Bonometti & Magnaudet37are shown by filled triangles. Figure 9: Boundary between peripheral and central breakup regions. The light yellow and dark yellow colours represent the regions for peripheral and central breakup. The corresponding data points from the present numerical simulation are shown as blue and black squares, respectively. Results of Bonometti & Magnaudet [37] are shown by filled triangles. Full size image We have now seen that a bubble that is initially spherical with a Ga and Eo corresponding to regions IV and V will breakup eventually. Does this mean that no single bubble can display a Ga and Eo corresponding to this region? The answer is a no. Large single bubbles have been created experimentally by many, see for example, refs 38 , 39 . It has been found in all of these studies that the stable shape for large-sized bubbles is a spherical cap. The initial conditions are extremely important for large bubbles, and experimenters take great care to generate an initial bubble which itself is in the form of a spherical cap. This is done by specially designed dumping cups. In fact ref. 39 note that only with a cup whose shape was very close to the final spherical cap bubble shape could they generate a stable bubble. Not just the curvature but particular care had to be taken to match the angle subtended by the cup shape at the centre of curvature to that of the final bubble shape, and to minimize external perturbations. In summary it was very difficult to create a single large spherical cap bubble since if these conditions were not enforced, the bubble would breakup and satellite bubbles were inevitably present in the wake. In addition, ref. 40 observes that in general spherical cap bubbles undergo tilting and wrinkling of their bottom, which results in the occasional peel off of satellite bubbles. The largest spherical cap bubbles that have been thus observed, to our knowledge, have Ga~10 4 and Eo~10 2 (ref. 39 ), which are well beyond the regime we have investigated. Batchelor [41] conducted a stability analysis of a steady rising spherical cap bubble to obtain an estimate of the largest stable bubble. This size is far smaller, and lies in regime V of our phase plot. These studies, and the computations of ref. 42 , underline the importance of initial conditions in this problem. In addition to spherical cap bubbles, toroidal bubbles too of much larger size have been experimentally observed by ref. 39 for different initial conditions and parameters. Our results show that a bubble that starts from a spherical shape has a vastly different fate, and can stay integral only when much smaller. Upward motion The vertical velocities of bubbles in the different regions is characterized in Fig. 10 . In region I, the vertical velocity monotonically increases and saturates at a terminal value. In region II, some minor oscillations are displayed initially owing to the skirt formation, but again a terminal velocity is reached. Region III displays oscillations of amplitude ~25% of the average velocity, but these were seen to quieten down somewhat once vortex shedding begins. Regions IV and V display irregular but large oscillations in the velocity. In both regions the oscillations are small at later times, but while in region IV, the final velocity is close to its maximum, in region V the upward movement of the centre of gravity of the dispersed phase has slowed down to about half its original velocity. This is because the bubble has disintegrated considerably in the latter case. 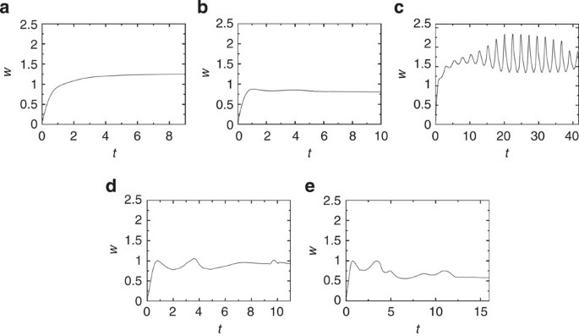Figure 10: Rise velocity for bubbles having markedly different dynamics. (a) region I: axisymmetric (Ga=10, Eo=1) (b) region II: skirted (Ga=10, Eo=200), (c) region III: zigzagging (Ga=70.7, Eo=1), (d) region IV: offset breaking up (Ga=70.7, Eo=20) and (e) region V: centrally breaking up bubble (Ga=70.7, Eo=200). In addition to the upward velocity, the in-plane components are unsteady too in regions III to V. Figure 10: Rise velocity for bubbles having markedly different dynamics. ( a ) region I: axisymmetric (Ga=10, Eo=1) ( b ) region II: skirted (Ga=10, Eo=200), ( c ) region III: zigzagging (Ga=70.7, Eo=1), ( d ) region IV: offset breaking up (Ga=70.7, Eo=20) and ( e ) region V: centrally breaking up bubble (Ga=70.7, Eo=200). In addition to the upward velocity, the in-plane components are unsteady too in regions III to V. Full size image The variation of dimensionless terminal velocity, w T versus Eo for different values of Ga is plotted in the Supplementary Fig. 8 . It can be seen that decreasing the value of Eo results in an increase in the terminal velocity for all values of Ga; however, as expected the rate of increase of the terminal velocity is higher for higher values of Ga. The bubbles that exhibit peripheral breakup (that is, bubbles lying in region IV in our phase plot, Fig. 1 ) tend to have an increase in their average rise velocity because of the presence of satellite bubbles [39] . We study the rise under gravity of an initially static and spherical bubble whose density and viscosity are fixed to be much smaller than that of the surrounding fluid. The parameters that govern the dynamics are the Galilee and the Eötvös numbers. Our extensive fully 3D study, with Ga and Eo ranging from 7 to 500 and 0.1 to 200, respectively, brings to light a number of features. We find five distinct regions in the phase plot, with sharply defined boundaries. The bubble is axisymmetric in region I, non-axisymmetric in regions II and III, and breaks in regions IV and V. Region II, where the bubble consists of an axisymmetric spherical cap and a skirt with minor asymmetries, is distinguished by the Mo ~10 −3 line from the dramatically asymmetrical bubbles of region III. This Morton number has been found in experiments to be the highest at which path instabilities are seen. Region II bubbles are non-oscillatory, whereas all bubbles of region III display path instabilities, in the form of spirals or zig-zags. This shows an intimate connection between shape and path asymmetries. In regions IV and V the bubble motion is unsteady and shows two different kinds of topology change: peripheral breakup and toroid formation, respectively, the latter is followed by breakup. Moving along lines of constant Morton number on this plot, that is, for bubbles of increasing radius placed in a given surrounding liquid, there are thus up to three transitions which take place. Some older experiments, for example, ref. 21 have given crude boundaries between different shapes of bubbles in regions I to III, with very good agreement with present simulations in the transition from axisymmetric to wobbly. At low Morton number in region IV, we show a new kind of bubble breakup, into a bulb-shaped bubble and a few satellite drops. Each transition is clearly distinguishable in terms of the completely different behaviour on either side. A maximum in kinetic plus surface energy occurs on the transition boundaries, a figure is provided in the Supplementary Material . The importance of studying this problem in 3D is brought out at many places in this paper. Other 3D studies have obtained the path instability, but not the transition to other regimes. We hope that our work will motivate experiments on initially spherical bubbles to check our phase plot. Formulation Three-dimensional simulation of a rising bubble (fluid ‘ i ') in a far denser and more viscous fluid (fluid ‘ o ’) under the action of buoyancy is considered, as shown in the Supplementary Fig. 1 . The bubble is assumed to be stationary at t =0. We use Cartesian coordinate system ( x , y , z ) to model the flow dynamics. Gravity acts in the negative z direction. Free-slip and no-penetration conditions are imposed on all the boundaries of the computational domain. A rising bubble undergoes an increase in volume as it rises, but for the vertical distances it travels in the present simulations, we may estimate a volume change of <0.5% for the air–water system. Thus, we assume the flow to be incompressible in the present study. The dimensional governing equations describing the flow dynamics are: where u =( u , v , w ) denotes the velocity field in which u , v and w represent the velocity components in the x , y and z directions, respectively, c is the volume fraction of the fluid in continuous phase (fluid ‘ i '), p is the pressure field, t denotes time. The density, ρ , and the viscosity, μ , are assumed to depend on the volume fraction of the fluid ‘ i ', c : where ρ i , μ i and ρ o , μ o are the density and dynamic viscosity of the dispersed and the continuous phases, respectively. In equation (2), F represents the combined body and surface forces per unit volume, which include the gravity and surface tension forces: where j denotes the unit vector along the vertical direction, σ and g represent the (constant) interfacial tension for the pair of fluids considered and gravitational acceleration, respectively, δ is the Dirac delta function (given by | ∇ c |), and κ = ∇ ˙ n is the interfacial curvature in which n is the outward-pointing unit normal to the interface. The following scaling is employed to render the governing equations dimensionless: where the velocity scale is , and the tildes designate dimensionless quantities. After dropping tildes from all non-dimensional variables, the governing dimensionless equations are given by where the dimensionless density and dynamic viscosity are given by Movies showing the bubble motion corresponding to Figs 5 and 10d,e can be found as Supplementary Materials . Numerical method A Volume-of-fluid (VOF) method with dynamic adaptive grid refinement based on the vorticity magnitude and bubble interface is used to simulate the bubble dynamics. A finite volume open source code, Gerris [43] is used that incorporates a height–function-based balanced force continuum surface force formulation for the inclusion of the surface force term in the Navier–Stokes equation [44] . A number of test cases have been performed by Popinet [45] to determine the order of errors in the surface force calculation as compared with other methods like combined level set and volume of fluid (CLSVOF), and front tracking. Gerris is able to minimize the amplitude of spurious currents, scaled with (2 R / σ ) 1/2 where σ is the surface tension coefficient, to <10 −12 as compared with other numerical simulations, which employed level-set (LS) [46] , CLSVOF [47] and front tracking [48] , which could go up to minimum amplitude of about 10 −6 . As shown in ref. 49 , Gerris performs best among other available numerical simulations for the problem of a damped small amplitude capillary wave, which makes it a good candidate for simulating surface tension-driven viscous flows. Also, a number of other test cases available in ref. 45 show that employed numerical method is state-of-the-art, and it is one of the best alternatives for simulating flows involving fluid–fluid interfaces. The effect of domain size and grid size has been tested to make sure that the results correspond to those for an unbounded domain and that they are free from numerical errors. The domain and grid independence tests are presented in the Supplementary Figs 2 and 3 , respectively. Supplementary Notes 1 and 2 contain a further justification of the domain and grid sizes used, respectively, in the present study. The numerical method has been well validated against theoretical results ( Supplementary Fig. 4 ; Supplementary Note 3 ) as well as experimental results ( Supplementary Figs 5 and 6 ; Supplementary Note 4 ). Characterization of bubble dynamics Assignment of a given bubble dynamics to a region is straightforward given that behaviour is so different on either side of each boundary. Bubbles which breakup and those which do not are clearly evident in visual examination of the time evolution of the shape. Similarly the difference between the two kinds of breakup (region IV–V) is very evident. The boundary between regions II and III is again evident by visual examination, since (a) the shapes are very different on either side of the boundary (b) the path in region II is oscillatory, whereas region III bubbles move up in a straight line. The green and blue colour in the phase plot ( Fig. 1 ) combine to give the region in the Ga–Eo plane where the bubble assumes an asymmetric shape. The asymmetry is computed as follows. The bubble is cut with eight vertical planes to get eight cross sections, each successive plane separated by an angle of π /8 rad. The area of a vertical face of each cross-section of the bubble is calculated and the percentage difference in the area with respect to a reference cross-section (lying in the y – z plane) is obtained. The root-mean-squared value of this data at each time step represents the degree of asymmetry, δ a . Because of the O (Δ x 2 ) scheme used in finite volume discretization, the error in calculation of area of cross-section( A ) may be estimated as where L v and L h are the bubble dimensions in the vertical and horizontal directions, in the cross-sectional plane. The errors in the bubble dimensions, Δ L v and Δ L h are of the order of the square of the smallest grid size, that is, 0.029 2 for a simulation with the coarsest mesh used in our study that is, Δ x =0.029. Thus we obtain Δ A / A ≈2 × 0.029 2 , or ≈0.0017 which is about 0.2%. The root-mean-squared error percentage is calculated for all the cross sections, which is denoted by δ a in this text. To be conservative, any variation within 0.5% in δ a is considered to represent a symmetric bubble, whereas the bubble is considered to be asymmetric when δ a exceeds 0.5%. As described in the main manuscript, shape asymmetry can be seen with or without an accompanying asymmetrical motion in the horizontal plane. The motion of the bubble is obtained by tracking the centre of gravity (centroid of the bubble) of the bubble with time. Our measure of deviations from azimuthal symmetry, δ a is for both kinds of asymmetry that is, oscillatory as well as non-oscillatory, whereas the centroid motion gives information about the deviation from vertical motion, that is, the path instability. The dashed lines in Fig. 1 are drawn between different regions to guide the eye. How to cite this article: Tripathi, M. K. et al. Dynamics of an initially spherical bubble rising in quiescent liquid. Nat. Commun. 6:6268 doi: 10.1038/ncomms7268 (2015).